Organic transistors with high thermal stability for medical applications The excellent mechanical flexibility of organic electronic devices is expected to open up a range of new application opportunities in electronics, such as flexible displays, robotic sensors, and biological and medical electronic applications. However, one of the major remaining issues for organic devices is their instability, especially their thermal instability, because low melting temperatures and large thermal expansion coefficients of organic materials cause thermal degradation. Here we demonstrate the fabrication of flexible thin-film transistors with excellent thermal stability and their viability for biomedical sterilization processes. The organic thin-film transistors comprise a high-mobility organic semiconductor, dinaphtho[2,3- b :2′,3′- f ]thieno[3,2- b ]thiophene, and thin gate dielectrics comprising a 2-nm-thick self-assembled monolayer and a 4-nm-thick aluminium oxide layer. The transistors exhibit a mobility of 1.2 cm 2 V −1 s −1 within a 2 V operation and are stable even after exposure to conditions typically used for medical sterilization. By taking full advantage of the mechanical flexibility and ruggedness that organic materials inherently possess, organic electronic devices are expected to open up possibilities for many new applications, such as flexible displays [1] , radio-frequency identification (RFID) tags [2] and large-area sensors [3] . Furthermore, the mechanical flexibility offered by organic electronics may enable the development of novel biomedical devices, such as large-area sensitive catheters [4] . However, if organic electronic devices are to be integrated into medical apparatuses, they must be able to withstand the sterilization conditions required to achieve asepsis and prevent infection, which usually involves exposure to temperatures in excess of 100 °C; typical sterilizing autoclaves operate in saturated steam at 121 °C. At such high temperatures, organic devices generally degrade, either as a result of the thermally induced oxidation of the organic semiconductor, or due to changes in the crystal structure or morphology of the thin films, or because of mechanical stresses induced by mismatches in the thermal expansion of the materials stack within the devices. The incorporation of organic electronic devices in biomedical applications will necessarily require a critical understanding and improvements of the thermal stability of these devices. One straightforward approach for fabricating thermally stable organic transistors involves the use of heat-resistant functional materials. Organic transistors that use pentacene as the organic semiconductor and heat-resistant polyimide as the gate dielectric, for example, retain their electronic functionality even after exposures to temperatures as high as 160 °C (ref. 5 ). However, these devices suffer from two limitations. First, the oxidization of pentacene to 6,13-pentacenequinone is dramatically accelerated at such high temperatures, and second, transistors with polyimide gate dielectrics usually require operation voltages of 20 V or higher, far exceeding the safety limit for medical applications. Recently, the operation voltages of organic transistors have been reduced to 3 V or less by utilizing high-capacitance gate dielectrics, such as high-permittivity metal oxides [6] , very thin organic insulating multilayers [7] and ionic gels [8] . Despite these advancements it remains challenging, however, to simultaneously achieve high thermal stability, low operation voltage and high field-effect mobility in flexible transistors that rely on smooth, ultra-thin, pinhole-free and thermally stable gate dielectrics. This study reports the fabrication of heat-resistant, flexible organic thin-film transistors (TFTs) that operate at voltages of 2 V and have a field-effect mobility of 1.2 cm 2 V −1 s −1 . The effects of exposing these TFTs to temperatures up to 160 °C were systematically investigated. We found that the heat-induced changes in the electrical performance of the TFTs are negligible for temperatures up to 120 °C, and that the device characteristics can be further stabilized by first annealing the TFTs at elevated temperatures before operation. The heat-resistant TFTs were realized using dinaphtho[2,3- b :2′,3′- f ]-thieno[3,2- b ]thiophene (DNTT) as the organic semiconductor [9] , [10] and a combination of a plasma-grown aluminium oxide (AlO x ) layer and an alkylphosphonic acid self-assembled monolayer (SAM) as the gate dielectric [11] . The effects of temperatures up to 160 °C on the crystal structure of the DNTT film and of temperatures up to 200 °C on the orientation of the alkylphosphonic acid molecules within the SAM were investigated using X-ray diffraction (XRD) and near-edge X-ray absorption fine structure (NEXAFS) spectroscopy, respectively. We found the SAM to be thermally stable over the temperature range explored; the ensemble-average tilt angles of C18-SAMs, for example, with respect to the surface normal changes only slightly (from 14° to 16°) on heating from room temperature to 160 °C. The practical applicability of heat-resistant organic TFTs was demonstrated by subjecting them to standard medical sterilization procedures, including heating to a temperature of 150 °C for 20 s in air. Under this condition, fluorescence microscopy showed that more than 92% of yeast cells plated on glass substrates are killed, whereas the changes in the transistor characteristics remain negligible. 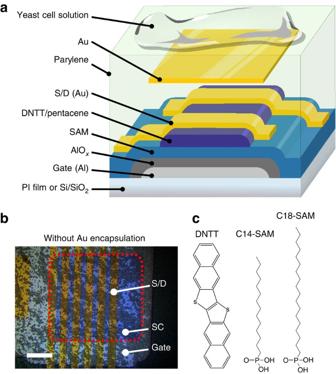Figure 1: Structure of the DNTT transistors. (a) Schematic cross-section of the transistors with parylene/Au encapsulation. The TFTs have a channel width of 500 μm and a channel length of 40 μm. (b) Photograph of a DNTT transistor covered with yeast cells. The dashed line represents the area of the semiconductor layer, and the scale bar indicates 200 μm. (c) Chemical structure of the organic semiconductor DNTT and the alkylphosphonic acid moleculesn-octadecylphosphonic acid (C18-SAM) andn-tetradecylphosphonic acid (C14-SAM) used for the self-assembled monolayers. Fabrication of heat-resistant flexible organic transistors Figure 1 shows a schematic of the cross-section ( Fig. 1a ) and a photograph ( Fig. 1b ) of the heat-resistant TFTs, which were fabricated with a thin AlO x /SAM gate dielectric on a flexible polyimide substrate. The chemical structures of DNTT and the alkylphosphonic acids ( n -tetradecylphosphonic acid, n -octadecylphosphonic acid) are shown in Fig. 1c . The TFTs were fabricated by depositing a 25-nm-thick aluminium layer as the gate electrode onto a 75-μm-thick polyimide substrate by thermal evaporation through a shadow mask. Transistors were also fabricated on oxidized silicon substrates for degradation studies and X-ray analysis. Oxygen-plasma treatment was performed to oxidize the surface of the thermally evaporated aluminium, resulting in a thin AlO x layer on the gate electrode. A plasma power of 100 W (for 10 min) was used to oxidize the aluminium surface on polyimide substrates, whereas a plasma power of 300 W (for 30 min) was used to oxidize the aluminium surface on silicon substrates. The substrates were subsequently dipped into a solution of 5-m M n -octadecylphosphonic acid or n -tetradecylphosphonic acid in isopropyl alcohol for 16 h to form a SAM with a thickness of about 2 nm (ref. 11 ). The combination of the AlO x and the SAM functions as the gate dielectric layer. Thirty-nm-thick DNTT or pentacene was then deposited by thermal evaporation to form the channel. Finally, 50-nm-thick Au was deposited by thermal evaporation through a shadow mask to define the source/drain contacts. The channel width and length of our TFTs were 500 and 40 μm, respectively. DNTT thin films for the XRD experiments were prepared under the same conditions, but without depositing Au on top. For the sterilization experiments, the transistors were encapsulated by sequentially depositing a 300-nm-thick layer of poly(chloro- para -xylylene), or parylene, by chemical vapour deposition, followed by a 200-nm-thick layer of gold and another 1-μm-thick parylene layer. Parylene was chosen as an encapsulation layer because of its biocompatibility, high thermal stability and low gas permeability [5] , [12] . After the fabrication process, the TFTs were annealed at temperatures according to the subsequent sterilization procedures. The annealing process (initial heating process) leads to an improved stability of the electrical TFT characteristics during the subsequent sterilization procedure. Figure 1: Structure of the DNTT transistors. ( a ) Schematic cross-section of the transistors with parylene/Au encapsulation. The TFTs have a channel width of 500 μm and a channel length of 40 μm. ( b ) Photograph of a DNTT transistor covered with yeast cells. The dashed line represents the area of the semiconductor layer, and the scale bar indicates 200 μm. ( c ) Chemical structure of the organic semiconductor DNTT and the alkylphosphonic acid molecules n -octadecylphosphonic acid (C18-SAM) and n -tetradecylphosphonic acid (C14-SAM) used for the self-assembled monolayers. Full size image In addition to the chemical stability of the organic semiconductor and the gate dielectric at elevated temperatures, good matching of the thermal expansion of the various materials within the device structure is another important requirement for heat-resistant devices. Given that the polyimide substrate has a small linear thermal expansion coefficient of 20 p.p.m. K −1 that is similar to that of aluminium (23.1 p.p.m. K −1 ), the expansion of these materials during exposure to elevated temperatures should not adversely affect the device performance. 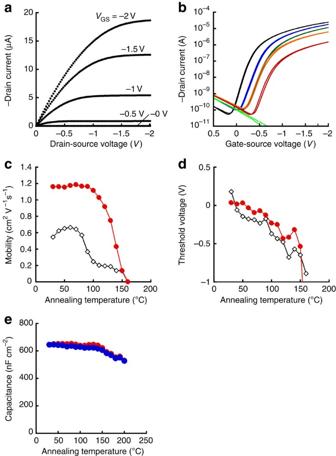Figure 2: Electrical properties of DNTT transistors. DC characteristics of a bare DNTT TFT are measured at room temperature before and after various thermal processes. (a) Output curves of a DNTT TFT before annealing. Gate-source voltages (VGS) were applied, changing from 0 to −2 V in steps of −0.5 V. (b) Transfer curves of a DNTT TFT after annealing in a nitrogen-filled glove box with <1 p.p.m. oxygen and moisture at different temperatures. A drain-source voltage (VDS) of −2 V was applied. For each measurement, the TFT was annealed at the indicated temperature and then allowed to cool to 30 °C for the measurement. Annealing temperatures were changed from 40°C to 170 °C. The black line represents a transfer curve obtained before annealing (at 30 °C). Other transfer curves were obtained at 30 °C after annealing at 100 (blue), 120 (dark green), 140 (orange), 150 (red), 160 °C (light green). (c) Field-effect mobility of DNTT (solid red circles) and pentacene (open black squares) TFTs as a function of annealing temperature. The mobilities were extracted from measurements performed at 30 °C. (d) Threshold voltage of DNTT (solid red circles) and pentacene (open black squares) TFTs as a function of annealing temperature. Note that incandd, solid circle represents data obtained from a DNTT TFT and open square from a pentacene TFT. (e) Capacitance of the aluminium oxide (AlOx)/octadecylphosphonic acid (SAM) gate dielectric sandwiched between an Al bottom electrode and a Au top electrode with changing annealing temperatures. Red circles represent the capacitance measured at each annealing temperature, while blue circles are the capacitance measured at room temperature after each annealing temperature. Although tetradecylphosphonic acid SAMs provide slightly larger field-effect mobility in organic transistors than octadecylphosphonic acid SAMs14, octadecylphosphonic acid SAMs were used in this experiment, since they were found to provide better thermal stability than tetradecylphosphonic acid SAMs. Thermal stability of the physical and electrical properties Figure 2 shows the electrical characteristics of the DNTT TFTs measured at 30 °C, before annealing. The effects of annealing were systematically evaluated by first measuring the electrical characteristics of the TFTs at 30 °C, followed by annealing at 40 °C for 30 min. The devices were then allowed to cool to 30 °C and measured. The same transistors were then annealed at 50 °C for 30 min, returned to 30 °C, and measured. This procedure was performed from 30 °C to 160 °C in steps of 10 °C. All of these experiments were carried out in a nitrogen-filled glove box with <1 p.p.m. each of oxygen and moisture. Figures 2a and 2b show the current–voltage characteristics of the organic TFTs. As can be seen, the on-state drain current ( I D ) at gate-source voltage ( V GS )=drain-source voltage ( V DS )=−2 V slightly decreases on annealing at 100 °C, due to a shift of the threshold voltage towards more negative values. This behaviour is consistent with our previous report [13] . Further annealing at temperatures above 150 °C for 30 min resulted in a degradation of the electrical performance. Figure 2e shows the capacitance of the AlO x /octadecylphosphonic acid (SAM) gate dielectric as a function of annealing temperature. The capacitance of the AlO x /SAM stack sandwiched between the Al bottom electrode and the Au top electrode indicates an excellent thermal stability of the gate dielectric up to temperatures of 150 °C, with a slight degradation on annealing beyond 160 °C. Figure 2: Electrical properties of DNTT transistors. DC characteristics of a bare DNTT TFT are measured at room temperature before and after various thermal processes. ( a ) Output curves of a DNTT TFT before annealing. Gate-source voltages ( V GS ) were applied, changing from 0 to −2 V in steps of −0.5 V. ( b ) Transfer curves of a DNTT TFT after annealing in a nitrogen-filled glove box with <1 p.p.m. oxygen and moisture at different temperatures. A drain-source voltage ( V DS ) of −2 V was applied. For each measurement, the TFT was annealed at the indicated temperature and then allowed to cool to 30 °C for the measurement. Annealing temperatures were changed from 40°C to 170 °C. The black line represents a transfer curve obtained before annealing (at 30 °C). Other transfer curves were obtained at 30 °C after annealing at 100 (blue), 120 (dark green), 140 (orange), 150 (red), 160 °C (light green). ( c ) Field-effect mobility of DNTT (solid red circles) and pentacene (open black squares) TFTs as a function of annealing temperature. The mobilities were extracted from measurements performed at 30 °C. ( d ) Threshold voltage of DNTT (solid red circles) and pentacene (open black squares) TFTs as a function of annealing temperature. Note that in c and d , solid circle represents data obtained from a DNTT TFT and open square from a pentacene TFT. ( e ) Capacitance of the aluminium oxide (AlO x )/octadecylphosphonic acid (SAM) gate dielectric sandwiched between an Al bottom electrode and a Au top electrode with changing annealing temperatures. Red circles represent the capacitance measured at each annealing temperature, while blue circles are the capacitance measured at room temperature after each annealing temperature. Although tetradecylphosphonic acid SAMs provide slightly larger field-effect mobility in organic transistors than octadecylphosphonic acid SAMs [14] , octadecylphosphonic acid SAMs were used in this experiment, since they were found to provide better thermal stability than tetradecylphosphonic acid SAMs. Full size image It is interesting to compare these results with those obtained for pentacene transistors, for which the device structure and the manufacturing process are nominally identical, except for the organic semiconductor. The mobility and threshold voltage of both the DNTT and pentacene TFTs are plotted as a function of annealing temperature in Fig. 2c and d , respectively. The mobility of the DNTT TFT is almost constant at 1.2 cm 2 V −1 s −1 for annealing temperatures up to ~100 °C, but shows a decrease on annealing beyond 100 °C. However, even after annealing at 120 °C the change in the mobility is <23%. In contrast, pentacene TFTs exhibit a substantial decrease in the mobility by 65% when annealed at 120 °C. This experiment demonstrates that DNTT transistors are much more stable at elevated temperatures compared with the quintessential pentacene transistors. The effects of annealing at elevated temperatures on the structure of the DNTT films were evaluated by XRD measurements using Cu-Kα X-ray radiation ( λ =1.541 Å). The out-of-plane and in-plane XRD spectra are shown in Fig. 3a and 3b , respectively, using a 2θ scanning range for the out-of-plane measurements from 3° to 10°, and from 15° to 35° for the in-plane measurements. The grazing angle of the in-plane measurement is 0.2° from the DNTT thin-film surface. The out-of-plane XRD spectra ( Fig. 3a ) show a single Bragg reflection peak at 2θ=5.5° and this Bragg reflection peak, corresponding to the (001) d-spacing of DNTT, appears at the same angle throughout the annealing process. This observation indicates that the lattice spacing in the direction perpendicular to the surface normal does not change with heating. In contrast to DNTT, pentacene undergoes a phase transition from its thin-film phase to its bulk phase at a temperature of 100 °C (ref. 14 ). The in-plane XRD spectra of DNTT ( Fig. 3b ), on the other hand, show three diffraction peaks. By comparison with X-ray crystallography of single-crystal DNTT [10] , [15] and pentacene [16] , which has a similar crystal structure to DNTT, we found that these three unique peaks in the in-plane XRD spectra correspond to the (110), (020) and (120) lattice planes of DNTT. The fact that we observe three sets of lattice planes that are nominally not parallel to each other in the in-plane spectra is a strong suggestion that our films are polycrystalline and that the DNTT grains are not preferentially oriented. The diffraction peaks at 2θ=23° and 27° in the in-plane XRD spectra were found to shift slightly towards larger diffraction angles on annealing above 100 °C, which corresponds to the temperature beyond which the electrical degradation of the DNTT TFTs sets in. The amounts by which the (001), (110), (020) and (120) diffraction peaks shift on annealing are plotted in Fig. 3c and 3d as a function of annealing temperature. From the measured shift of the diffraction peaks in the in-plane XRD spectra, the change of the lattice constants on annealing can be estimated. In particular, the lattice constant along the a axis increases by 1.5% from 6.10 Å to 6.19 Å on annealing at 160 °C. On the other hand, the lattice constant along the b axis decreases only slightly by 0.65% from 7.77 Å to 7.72 Å, while the lattice spacing along the c axis decreases negligibly by 0.3% from 16.36 Å to 16.31 Å on annealing at 160 °C. The observed reduction in the field-effect mobility (from initially 1.2 to 0.4 cm 2 V −1 s −1 after annealing at 140 °C) is thus attributed to changes in the crystal structure of the DNTT film brought about by the following two mechanisms. One is a phase transition induced at 100 °C, which reduces the conductivity within the grains (not unlike pentacene [5] , but at higher temperature). The other is a change in the shape of the grains, which reduces the contacts between neighbouring grains. Evidence to support the latter mechanism was found from atomic force microscopy observations of the DNTT morphology, which revealed that after annealing at 140 °C the film roughens significantly and features as tall as 300 nm begin to emerge ( Supplementary Fig. S1 ). 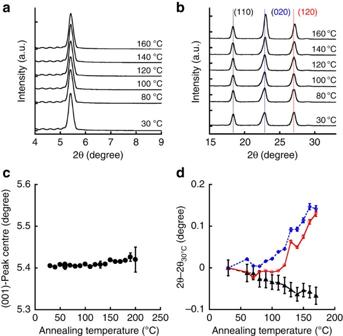Figure 3: XRD spectra of DNTT films. The structure for XRD characterizations is a 30-nm-thick DNTT film deposited on AlOx/SAM layers. Samples have no encapsulation and oxidized silicon substrates are used. The XRD measurements were carried out at room temperature. (a) Out-of-plane XRD spectra of a DNTT film before and after annealing. Annealing temperatures are shown on each spectrum in the graph. (b) In-plane XRD spectra of a DNTT film before and after annealing. The peaks at 18°, 23° and 27° correspond to the (110), (020) and (120) lattice planes, respectively. Annealing temperatures are shown on each spectrum in the graph. (c) Diffraction angle of the (001) peak obtained from the out-of-plane XRD spectra as a function of annealing temperature. (d) Diffraction angles of the (110) (black), (020) (blue) and (120) (red) peaks obtained from the in-plane XRD spectra as a function of annealing temperature. Error bars incanddrepresent standard errors from regression analysis to detect centres of diffraction peaks. a.u., arbitrary unit. Figure 3: XRD spectra of DNTT films. The structure for XRD characterizations is a 30-nm-thick DNTT film deposited on AlO x /SAM layers. Samples have no encapsulation and oxidized silicon substrates are used. The XRD measurements were carried out at room temperature. ( a ) Out-of-plane XRD spectra of a DNTT film before and after annealing. Annealing temperatures are shown on each spectrum in the graph. ( b ) In-plane XRD spectra of a DNTT film before and after annealing. The peaks at 18°, 23° and 27° correspond to the (110), (020) and (120) lattice planes, respectively. Annealing temperatures are shown on each spectrum in the graph. ( c ) Diffraction angle of the (001) peak obtained from the out-of-plane XRD spectra as a function of annealing temperature. ( d ) Diffraction angles of the (110) (black), (020) (blue) and (120) (red) peaks obtained from the in-plane XRD spectra as a function of annealing temperature. Error bars in c and d represent standard errors from regression analysis to detect centres of diffraction peaks. a.u., arbitrary unit. Full size image The thermal stability and the electrical performance of gate dielectrics comprising a thin plasma-grown AlO x layer and an alkylphosphonic acid SAM were evaluated from measurements on capacitors consisting of a 20-nm-thick Al bottom electrode, a 4-nm-thick AlO x layer, a 2-nm-thick SAM and a 50-nm-thick Au top electrode. The molecular structure of the adsorbed SAM was also examined by NEXAFS spectroscopy before the deposition of the Au top electrodes. We found that the capacitance of the AlO x /SAM dielectric is stable up to a temperature of 150 °C, but decreases from 809 to 641 nF cm −2 on annealing at 160 °C. This decrease in capacitance may be the reason for the observed reduction of the on-state drain current by 21%, as seen in Fig. 2 . Furthermore, NEXAFS spectroscopy was used to examine the molecular orientation and stability of the SAM at elevated temperatures. 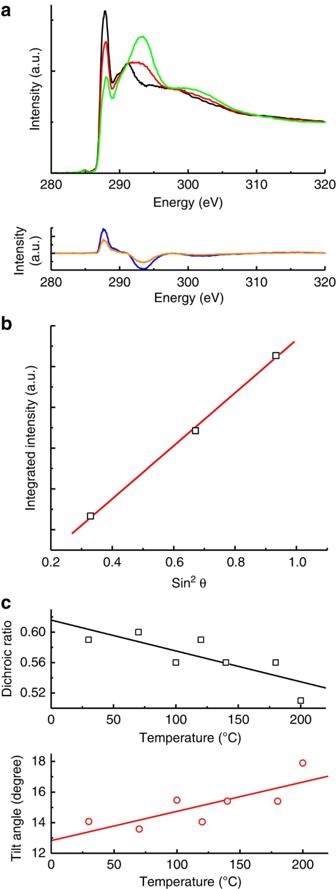Figure 4: NEXAFS partial electron yield spectra ofn-octadecylphosphonic acid SAM. Samples measured in these experiments were structured as AlOx/SAM on oxidized silicon substrates without organic semiconductors, metal electrodes or encapsulation layers. (a) The upper panel gives representative NEXAFS partial electron yield spectra acquired at the carbon K-edge of ann-octadecylphosphonic acid SAM for X-ray incident angles of 75° (black), 55° (red) and 35° (green). The lower panel shows the differences between the spectra measured at 75° and 35° (blue) and between the spectra measured at 55° and 35° (orange). Data are pre- and post-edge normalized. (b) Extracted 1 s to σ* integrated intensity of C–H bonds from the spectra shown inaas a function of X-ray incident angles. (c) Dichroic ratio and average tilt angles from the surface normal as a function of temperature for ann-octadecylphosphonic acid SAM annealed at different temperatures. The straight lines inbandcare guides to the eye. a.u., arbitrary unit. Figure 4a shows the NEXAFS spectra of a representative C18-SAM annealed at 70 °C, at different X-ray incident angles of 75°, 55° and 35°. The spectra show the C1s to σ* transitions attributed to C–H bonds at 287.8 eV, and the C1s to σ* transitions attributed to C–C bonds at 293.5 and 302.6 eV. The extent of the preferential orientation of the alkylphosphonic molecules in the SAMs can be quantified by examining the integrated intensity of the σ* C–H resonance at 287.8 eV. Figure 4b summarizes the resulting integrated intensity of the first angle-dependent σ* C–H resonance as a function of X-ray incident angle. A series of the row data can be seen in Supplementary Fig. S2 . As shown in Fig. 4c , the analysis yielded a dichroic ratio (DR) value of 0.5–0.6 for C18-SAMs that suggests that the alkylphosphonic acid molecules within the SAM are oriented with their chains preferentially upright with respect to the substrate; this degree of preferential orientation indicated by the DR is among the highest reported for SAMs. Furthermore, we found that this preferential orientation of the alkylphosphonic acid molecules is maintained up to a temperature of 200 °C, confirming the excellent thermal stability of these SAMs. Analysis with the Building Block Model indicates that C18-SAMs are tilted with an angle of 13° to 18° from the surface normal, and this tilt angle is largely preserved on thermal annealing at elevated temperatures. Additional technical details about the NEXAFS analysis are given in the Methods and Supplementary Methods . Figure 4: NEXAFS partial electron yield spectra of n -octadecylphosphonic acid SAM. Samples measured in these experiments were structured as AlO x /SAM on oxidized silicon substrates without organic semiconductors, metal electrodes or encapsulation layers. ( a ) The upper panel gives representative NEXAFS partial electron yield spectra acquired at the carbon K-edge of an n -octadecylphosphonic acid SAM for X-ray incident angles of 75° (black), 55° (red) and 35° (green). The lower panel shows the differences between the spectra measured at 75° and 35° (blue) and between the spectra measured at 55° and 35° (orange). Data are pre- and post-edge normalized. ( b ) Extracted 1 s to σ* integrated intensity of C–H bonds from the spectra shown in a as a function of X-ray incident angles. ( c ) Dichroic ratio and average tilt angles from the surface normal as a function of temperature for an n -octadecylphosphonic acid SAM annealed at different temperatures. The straight lines in b and c are guides to the eye. a.u., arbitrary unit. Full size image Medical sterilization procedures on organic transistors Typical medical sterilization occurs by thermal processes, for example, 150 °C for 20 s with moisture at an atmospheric pressure. The practical applicability of our heat-resistant flexible organic transistors for medical instruments and their ability to simultaneously offer high thermal stability, mechanical flexibility and sustained electrical performance was demonstrated by subjecting the TFTs to typical sterilization treatments at temperatures up to 150 °C. We also carried out sterilization with boiling water at 100 °C or with longer-time heating at 121 °C for 20 min, or 100 °C for 30 min under atmospheric pressure. We encapsulated organic transistors with parylene and Au encapsulation to protect them against water exposure. The influence of parylene encapsulation on the thermal stability of the TFTs is shown in Supplementary Fig. S3 . To quantify the effect of medical sterilization procedures on the electrical characteristics of organic TFTs, we subjected yeast cells (on glass substrates) and organic TFTs (on flexible polyimide) simultaneously to sterilization in boiled water for 30 min and to various heat treatments at temperatures above 100 °C in air. The electrical characteristics of the organic TFTs were measured before and after the sterilization procedures ( Fig. 5 ). The effect of other sterilization procedures can be seen in Supplementary Fig. S4 . The total density of the yeast cells, as well as the density of dead cells, was measured with a sample on a glass substrate before and after the sterilization process using fluorescence microscopy ( Fig. 5a–f ). 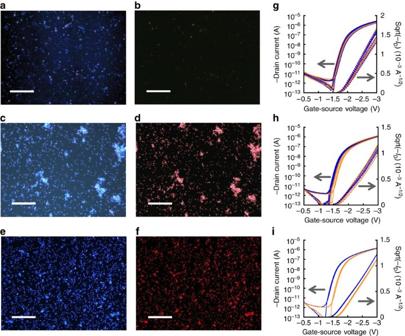Figure 5: Fluorescence microscopy images and TFT transfer curves before and after sterilization experiments. (a) Fluorescence microscopy images showing the total density of yeast cells and (b) the density of dead cells before sterilization as control sample without any heating. (c) Fluorescence microscopy images showing the total density of yeast cells and (d) the density of dead cells after sterilization at 150 °C for 20 s in air. (e) Fluorescence microscopy images showing the total density of yeast cells and (f) the density of dead cells after heat treatment at 121 °C for 20 min in air. Scale bars indicate 200 μm. (g) Transfer curves of a DNTT TFT before (blue line) and after (orange line) immersion in boiling water (100 °C) for 30 min; (h) before and after heat treatment at a temperature of 150 °C; and (i) before and after heat treatment at a temperature of 121 °C for 20 min in air. Right axis labels ing–iare square root of drain current (ID). The sterilization experiments were carried out in the air. The fluorescence microscopy experiments were carried out on glass substrates, and the TFTs were fabricated on flexible polyimide. Figure 5: Fluorescence microscopy images and TFT transfer curves before and after sterilization experiments. ( a ) Fluorescence microscopy images showing the total density of yeast cells and ( b ) the density of dead cells before sterilization as control sample without any heating. ( c ) Fluorescence microscopy images showing the total density of yeast cells and ( d ) the density of dead cells after sterilization at 150 °C for 20 s in air. ( e ) Fluorescence microscopy images showing the total density of yeast cells and ( f ) the density of dead cells after heat treatment at 121 °C for 20 min in air. Scale bars indicate 200 μm. ( g ) Transfer curves of a DNTT TFT before (blue line) and after (orange line) immersion in boiling water (100 °C) for 30 min; ( h ) before and after heat treatment at a temperature of 150 °C; and ( i ) before and after heat treatment at a temperature of 121 °C for 20 min in air. Right axis labels in g – i are square root of drain current ( I D ). The sterilization experiments were carried out in the air. The fluorescence microscopy experiments were carried out on glass substrates, and the TFTs were fabricated on flexible polyimide. Full size image To confirm that this temperature is sufficient for sterilization, we first put yeast bacteria onto a glass surface and applied two different dyes to stain our yeast culture: 4′,6-diamidino-2-phenylindole (DAPI), which stains all yeast cells and fluoresces in the blue when excited with ultraviolet light; and propidium imide, which preferentially stains dead cells and fluoresces in the red when excited with green light. Figure 5a–f shows the fluorescence microscopy images acquired under ultraviolet and green light irradiation before and after sterilization at 150 °C for 20 s or at 121 °C for 20 min in air. Quantification of the fluorescent intensities indicates that 93% of the yeast cells are killed on sterilization at 150 °C (note that the fluorescence experiments were performed on glass substrates, rather than directly on the flexible TFTs, as the background fluorescence from the polyimide, the DNTT and the parylene would interfere with the fluorescence measurements.). Having verified the effectiveness of this sterilization treatment in killing yeast cultures, we subjected the flexible DNTT TFTs to the same treatment (150 °C for 20 s in air) as well as to saturated steam for 20 min and to boiling water for 30 min. Figure 5g–i shows that the on-state drain current (1.2 μA) and the on/off ratio (8×10 5 ) are practically unaffected by these sterilization procedures. More details can be seen in Supplementary Fig. S5 . The orientation of the alkylphosphonic acid molecules in the SAM, as extracted from DR analysis or tilt-angle estimation, naturally depends on the molecule chemistry, the roughness of the substrates and the details of the SAM preparation conditions. Compared with SAMs based on alkylsilanes [17] , [18] , [19] , the use of alkylphosphonic acids is known to offer better stability and a smaller tendency for homo-condensation. In addition, alkylphosphonic acid SAMs exhibit more favourable molecular orientation, as evidenced by the larger DR. For comparison, SAMs comprising alkylthiols adsorbed on gold, for example, were consistently found to exhibit a DR of 0.4. Adsorption of n -phenylthiolates on polycrystalline gold and single-crystalline GaAs from ethanol yields a DR of 0.3–0.4; deposition of the same compounds from a mixture of ethanol and tetrahydrofuran results in negligible adsorption and a DR near 0 (ref. 20 ). In contrast, the DR of our C18-SAMs is in the range of 0.5–0.6. These values rival those measured for thin layers of pentacene adsorbed on polycrystalline gold and silicon dioxide surfaces [21] , which is surprising given the rigidity of pentacene and the relative floppiness of alkyl chains. In addition to the superior electrical stability of the transistors with AlO x /SAM gate dielectric, the DR of alkylphosphonic acid SAMs remains above 0.4 even after annealing at a temperature of 160 °C. Similar to alkylthiol SAMs [22] , the thermal stability of alkylphosphonic acid SAMs can be further improved by choosing the optimum length of the alkyl chains [14] , making alkylphosphonic acid SAMs a promising choice for the gate dielectric in heat-resistant low-voltage transistors. In conclusion, we have demonstrated heat-resistant, flexible, organic TFTs that are able to withstand the harsh conditions during medical sterilization treatments. Both the organic semiconductor DNTT and the alkylphosphonic acids that serve as part of the high-capacitance gate dielectric are commercially available. Although the unique combination of these materials is important, the TFT fabrication process also has a critical role in optimizing performance and stability. For example, the deposition of a smooth aluminium gate electrode is a crucial prerequisite for the formation of a dense, pinhole-free gate dielectric. While the semiconductor utilized in this work is deposited in vacuum, soluble derivatives that are compatible with printing or other solution-based processes are also available [23] , [24] . Further improvements in field-effect mobility will be possible by printing inorganic semiconducting nanowires or nano-ribbons [25] . Materials The molecules n -octadecylphosphonic acid or n -tetradecylphosphonic acid were used to form SAMs on plasma-grown AlO x as the dielectric. For cell staining, DAPI (-Cellstain-DAPI solution) and 3,8-diamino-5-[3-(diethylmethylammonio)propyl]-6-phenylphenanthridinium diiodide (propidium imide: -Bacstain-PI solution) from Dojindo Lab were used. NEXAFS measurements The NEXAFS experiments were carried out at the NIST/DOW soft X-ray materials characterization facility located at beam line U7A at the National Synchrotron Light Source at Brookhaven National Laboratories. Partial electron yield NEXAFS spectra were acquired at the carbon K-edge, normalized by the corresponding incident beam intensity, and the spectra were subsequently pre- and post-edge normalized [20] , [26] , [27] . Given the applied bias, the partial electron yield detector is only sensitive to Auger electrons emitting from the top 2 nm (ref. 28 ). The ensemble-average preferential orientation of the molecules within the SAMs can be quantitatively assessed by examining the variations in the integrated intensity associated with the 1 s to σ* transitions of the C–H bonds as function of X-ray incident angles, 75°, 55° and 35°. The resonance intensities vary with the X-ray incident angles: specifically, the σ* C–H resonances grow while the σ* C–C resonances diminish with increasing incident angles. This phenomenon, where the σ* C–H resonances grow at the expense of the σ* C–C resonances, is a strong indication that the molecules at the film surface are preferentially oriented with their chains upright with respect to the substrate. The contributions from the isotropic background and the step edge were eliminated by subtracting two original spectra (any two) that had been pre- and post-edge normalized. This process eliminates the isotropic contributions to the NEXAFS spectra and isolates the angle-dependent resonances to show three distinct angle-dependent resonances. Three peaks at 287.8, 293.5 and 302.6 eV were identified from the different spectra. This positive slope verifies that the molecules are preferentially oriented in the upright position with respect to the substrate. Specifically, the DR was extracted from the integrated intensities of the 1 s to σ* resonance, attributed to C–H bonds, at the different incident angles according to equation 1 below: where I is the integrated intensity of the 1 s to σ* resonance as a function of incident angle. DR can vary from −1 to +0.75 (refs 17 , 29 ), with a more positive value for the C–H σ* plane corresponding to a smaller average tilt angle from the substrate normal. Similar calculations were done for all the samples, that is, a C18-SAM and a C14-SAM on AlO x annealed at different temperatures. The top figure in Fig. 4c displays the DR of the C18-SAM annealed at different temperatures, and the solid line represents a linear fit that reveals the temperature dependence of DR. Fitting the data obtained in this study to the Building Block Model for spinning chains yields the ensemble-average tilt angle between the molecular axis and the substrate normal [26] , [27] , [30] , [31] . Figure 4c also displays the tilt angles for the C18-SAM annealed at different temperatures. Parylene encapsulation An encapsulation layer has to meet at least the following four criteria: low gas permeability, especially for oxygen and water; minimum damage inflicted on the organic semiconductor layer during the deposition; suppression of the volatility of the organic semiconductor molecules at elevated temperatures; and biocompatibility (optional). For these reasons we have chosen parylene to encapsulate our TFTs. Although parylene has proven useful to encapsulate pentacene transistors [12] , [13] , this is the first demonstration of parylene encapsulation for DNTT TFTs with SAM-based gate dielectrics, which was crucial to simultaneously achieve high mobility (1.2 cm 2 V −1 s −1 ) and high thermal stability (150 °C). Medical sterilization is typically performed in saturated steam or boiling water. Under these conditions, a single parylene layer does not provide sufficient protection of the organic TFTs. We have therefore encapsulated the TFTs with a triple-layer stack of 300-nm-thick parylene, 200-nm-thick Au and 1-μm-thick parylene. The thickness of the first parylene layer (300 nm) is a compromise, as it was found that thinner layers provide insufficient protection of the organic semiconductor layer during the subsequent Au deposition, while thicker layers lead to a lateral penetration of gases along the parylene layer [12] . Electrical measurements For the measurements of the electric characteristics of the TFTs, a semiconductor parameter analyzer (4155C, Agilent) was used. A precision LCR meter (4284A, Agilent) was used to measure the capacitance. For the XRD measurement, a high-resolution X-ray diffraction system (SmartLab, Rigaku) was used. To image the surface of the organic semiconductor layers we used a contact-mode atomic force microscope (AFM, NanoScope IIIa, Veeco Instruments). An inverted Metallurgical Microscope (GX71; Olympus) equipped with a light source (U-RFL-T, Olympus) was used in the fluorescence microscopy experiments. How to cite this article: Kuribara, K. et al . Organic transistors with high thermal stability for medical applications. Nat. Commun. 3:723 doi: 10.1038/ncomms1721 (2012).